The quantum nature of skyrmions and half-skyrmions in Cu2OSeO3 The Skyrme-particle, the skyrmion, was introduced over half a century ago in the context of dense nuclear matter. But with skyrmions being mathematical objects—special types of topological solitons—they can emerge in much broader contexts. Recently skyrmions were observed in helimagnets, forming nanoscale spin-textures. Extending over length scales much larger than the interatomic spacing, they behave as large, classical objects, yet deep inside they are of quantum nature. Penetrating into their microscopic roots requires a multi-scale approach, spanning the full quantum to classical domain. Here, we achieve this for the first time in the skyrmionic Mott insulator Cu 2 OSeO 3 . We show that its magnetic building blocks are strongly fluctuating Cu 4 tetrahedra, spawning a continuum theory that culminates in 51 nm large skyrmions, in striking agreement with experiment. One of the further predictions that ensues is the temperature-dependent decay of skyrmions into half-skyrmions. Skyrmionic spin textures in magnetic materials correspond to magnetic topological solitons. They were first observed in the non-centrosymmetric B20 helimagnets MnSi [1] , [2] , FeGe [3] and Fe 0.5 Co 0.5 Si (ref. 4 ). These skyrmionic textures are encountered also in a completely different branch of physics: in the theoretical description of nuclear matter [5] , [6] . In this setting the skyrmions are of course not related to magnetic degrees of freedom, but rather to particles emerging from cold hadron vector fields at densities a few times that of ordinary nuclear matter. This is the density range relevant for compact astronomical objects such as neutron stars [7] , [8] , [9] . The perhaps perplexing connection between these two seemingly disparate fields of physics is borne out of the underlying mathematical structures [7] , [8] , [9] , [10] , [11] , [12] , [13] , [14] . The physical phenomena in the two different settings are both governed by an emerging set of differential equations with topological solitonic solutions: the skyrmions found first by Skyrme in the 1960s (ref. 5 ). In this context, we investigate the formation and microscopic origin of the observed magnetic skyrmions in helimagnets. These skyrmions are large objects compared with the atomic length scale: they are about three orders of magnitude larger in size than the interatomic lattice spacing. Understanding the origin of these nanometre-scale skyrmions therefore requires a multi-scale approach. In the above-mentioned B20 helimagnets, such is however not viable because all these materials are metallic. The metallicity causes low-energy, delocalized electronic and magnetic degrees of freedom to mix so that they intrinsically involve multiple energy and spatial scales, which renders a multi-scale approach presently intractable. This is very different in the recently discovered skyrmionic material Cu 2 OSeO 3 , a large band-gap Mott insulator. The band gap enforces a natural separation between electronic and magnetic energy scales, which is advantageous for theoretical studies, as it allows for an accurate multi-scale approach. Cu 2 OSeO 3 is actually the first example of an insulating material displaying the chiral helimagnetism that is desired for skyrmion formation while sharing the non-centrosymmetric cubic space group P 2 1 3 of the metallic B20 phases, but with a unit cell that is much more complex, containing 16 Cu atoms. Due to the presence of a magnetoelectric coupling [15] , [16] , its skyrmions can be manipulated by an electric field [17] , [18] , [19] , which is in principle very energy efficient as this avoids losses due to joule heating. Here we present the results of a quantitative multi-scale study of Cu 2 OSeO 3 , from the atomic up to the mesoscopic length scale. We find that the chiral helimagnetism and skyrmion formation in Cu 2 OSeO 3 relies on the presence of Cu 4 tetrahedral building blocks that have a strong quantum-mechanical character. These effective entities spawn a continuum theory that results in skyrmions with a diameter of 51 nm, in quantitative agreement with reported experiments [15] , and lead to a series of key experimental ramifications. Most notably, a skyrmion fractionalization in a specific temperature and magnetic field range, the existence of weakly dispersive magnetic excitations at high energies, and the presence of a weak antiferromagnetic indentation of the primary ferrimagnetic order parameter, which turns out to be responsible for the sign of the magnetic chirality. The quantum nature of the tetrahedral building blocks is also responsible for the reduction of the local spin expectation values and the low effective energy scale (which sets, for example, the value of the ordering temperature T C ), compared with the microscopic exchange energy scales. Roadmap of multi-scale approach The key aspects of helimagnetism and skyrmion formation in chiral magnetic systems such as Cu 2 OSeO 3 are shown in Fig. 1 and the main steps of our multi-scale approach are outlined in Fig. 2 . We first evaluate the Heisenberg exchange and Dzyaloshinskii-Moriya (DM) interactions at the atomic level, using ab initio density functional theory (DFT) calculations ( Fig. 2a ). The resulting parameters reveal a striking separation of exchange energy scales which split the system into a network of magnetically ‘weak’ and ‘strong’ tetrahedra ( Supplementary Note 1 ). The latter are the basic building blocks of helimagnetism in Cu 2 OSeO 3 : each ‘strong’ tetrahedron behaves as a spin-1 triplet (apart from a finite quintet admixture, see Methods section), protected by a large energy gap of Δ ≃ 275 K ( Fig. 2c ). Integrating out the dominant energy scale leads to an effective model on the so-called trillium lattice ( Fig. 2d ), marking a close analogy to MnSi and FeGe. The description at the mesoscopic scale is finally achieved by a long-wavelength expansion of the effective model, which delivers the two basic parameters that control the skyrmionic physics ( Fig. 1 ) in Cu 2 OSeO 3 : the exchange stiffness and the twisting parameter . Supplementing the free energy with further anisotropies and entropic effects, and using a minimal amount of experimental information, we arrive at a quantitative Dzyaloshinskii model, which in turn gives access to the magnetic phase diagram and other experimentally accessible observables. The ensuing notable predictions are the presence of a fractionalized skyrmion phase ( Fig. 1c ), the presence of a small AFM canting, which is adiabatically tied to the twisting of the total magnetization ( Fig. 1e,f ), and the important role of the canting in controlling the sign of the magnetic chirality. The quantum-mechanical nature of the ‘strong’ tetrahedra also has an additional number of profound ramifications that will be discussed in detail. 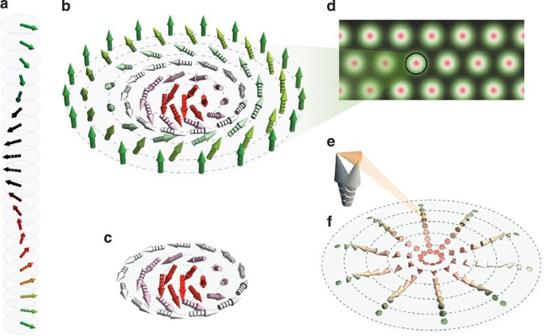Figure 1: Spin textures in chiral helimagnets. Besides flat helices (a), chiral helimagnets like Cu2OSeO3manifest radially symmetric topological solitons like skyrmions (b) or half-skyrmions (c), where the local order parameter (sectioned arrows) forms a double-twisted core, tracing out the whole (b) or half (c) of the Bloch sphere. (d) Parallel skyrmions can form densely packed lattices in two spatial dimensions. Ina, the colouring of the sectioned arrows tracks the direction of the magnetization in the plane of rotation, while in (b–d) it tracks the longitudinal magnetization. (e) Quantitative first-principles calculations predict that the ferrimagnetic order in Cu2OSeO3is locally altered by the multi-sublattice structure, leading to weak antiferromagnetism (depicted by orange arrowheads). (f) The skyrmion texture is locally composed of these three-dimensional canted spin patterns. Thus, the weak antiferromagnetic order itself is modulated along with the primary ferrimagnetic twisting shown inb. Figure 1: Spin textures in chiral helimagnets. Besides flat helices ( a ), chiral helimagnets like Cu 2 OSeO 3 manifest radially symmetric topological solitons like skyrmions ( b ) or half-skyrmions ( c ), where the local order parameter (sectioned arrows) forms a double-twisted core, tracing out the whole ( b ) or half ( c ) of the Bloch sphere. ( d ) Parallel skyrmions can form densely packed lattices in two spatial dimensions. In a , the colouring of the sectioned arrows tracks the direction of the magnetization in the plane of rotation, while in ( b – d ) it tracks the longitudinal magnetization. ( e ) Quantitative first-principles calculations predict that the ferrimagnetic order in Cu 2 OSeO 3 is locally altered by the multi-sublattice structure, leading to weak antiferromagnetism (depicted by orange arrowheads). ( f ) The skyrmion texture is locally composed of these three-dimensional canted spin patterns. Thus, the weak antiferromagnetic order itself is modulated along with the primary ferrimagnetic twisting shown in b . 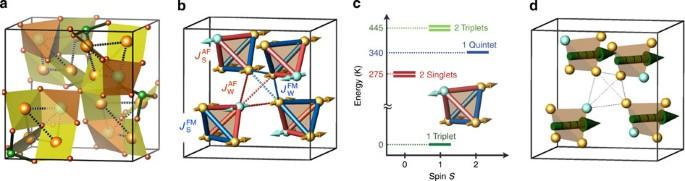Figure 2: Multi-scale modelling of Cu2OSeO3. (a) The crystal structure is shaped by Cu(2)O4plaquettes (yellow) and Cu(1)O5bipyramids (orange), and covalent Se-O bonds (thick lines), forming a sparse three-dimensional lattice. This lattice can be tiled into tetrahedra (dashed lines), each composed of one Cu(1) and three Cu(2) sites, depicted by large light brown and light cyan spheres, respectively. (Smaller spheres show the remaining non-magnetic sites). (b) The magnetic Cu2+ions form a distorted pyrochlore lattice, a network of corner-shared tetrahedra. DFT calculations evidence the presence of both types of magnetic interactions—antiferromagnetic (red) and ferromagnetic (blue), in agreement with experimental magnetic structure (arrows). The strength of a certain coupling is indicated by the thickness of the respective line. The strongest couplings,and, are found within the tetrahedra (shaded), while the couplings between the tetrahedra,,, and(the latter is a longer-range coupling), are substantially weaker (dashed lines). (c) The quantum-mechanical treatment of a single tetrahedrontyields a magnetic spinSt=1 ground state, separated from the lowest lying excitation by a large gap Δ≃275 K. (d) The tetrahedra reside at the vertices of a trillium lattice, exactly like the Mn ions in MnSi. The quantum-mechanical nature of the effective moments is indicated by sectioned arrows. Full size image Figure 2: Multi-scale modelling of Cu 2 OSeO 3 . ( a ) The crystal structure is shaped by Cu(2)O 4 plaquettes (yellow) and Cu(1)O 5 bipyramids (orange), and covalent Se-O bonds (thick lines), forming a sparse three-dimensional lattice. This lattice can be tiled into tetrahedra (dashed lines), each composed of one Cu(1) and three Cu(2) sites, depicted by large light brown and light cyan spheres, respectively. (Smaller spheres show the remaining non-magnetic sites). ( b ) The magnetic Cu 2+ ions form a distorted pyrochlore lattice, a network of corner-shared tetrahedra. DFT calculations evidence the presence of both types of magnetic interactions—antiferromagnetic (red) and ferromagnetic (blue), in agreement with experimental magnetic structure (arrows). The strength of a certain coupling is indicated by the thickness of the respective line. The strongest couplings, and , are found within the tetrahedra (shaded), while the couplings between the tetrahedra, , , and (the latter is a longer-range coupling), are substantially weaker (dashed lines). ( c ) The quantum-mechanical treatment of a single tetrahedron t yields a magnetic spin S t =1 ground state, separated from the lowest lying excitation by a large gap Δ ≃ 275 K. ( d ) The tetrahedra reside at the vertices of a trillium lattice, exactly like the Mn ions in MnSi. The quantum-mechanical nature of the effective moments is indicated by sectioned arrows. Full size image Description at the atomic level To elucidate the quantum origin of the skyrmion textures in Cu 2 OSeO 3 , we proceed with a calculation of magnetic interactions at the atomic level. In undoped cuprates with Cu 2+ atoms, such as Cu 2 OSeO 3 , the localized S =1/2 magnetic degrees of freedom originate from a single hole in the 3 d electronic shell. In the crystal structure of Cu 2 OSeO 3 , the Cu 2+ atoms make up a three-dimensional network of corner-sharing tetrahedra ( Fig. 2b ) with two inequivalent Cu sites, Cu(1) and Cu(2) featuring a different local environment: Cu(1)O 5 bipyramids and distorted Cu(2)O 4 plaquettes, respectively [20] , [21] . Each tetrahedron contains Cu(1) and Cu(2) in a ratio of 1:3. The resulting net of magnetic Cu ions in Cu 2 OSeO 3 thus has a structure that is rather different from the previously mentioned metallic B20 helimagnets such as MnSi, where the magnetic Mn ions form a three-dimensional corner-sharing net of triangles, commonly referred to as the trillium lattice. The more complex crystal structure of Cu 2 OSeO 3 leads to five inequivalent superexchange coupling constants J ij between neighbouring S =1/2 copper spins i and j (see Supplementary Fig. 1 ) and also five different Dzyaloshinskii–Moriya (DM) vectors D ij in the microscopic magnetic Hamiltonian where S i denotes the quantum-mechanical spin operator at the Cu site i . We have determined these coupling constants ( Table 1 ) by means of an extended set of ab initio density-functional-based electronic structure calculations. As our numerical estimates are substantially higher than the values reported in the literature [22] , they were cross-checked by calculating the magnetic ordering temperature T C and the T dependence of magnetization and magnetic susceptibility by means of large-scale Quantum Monte Carlo (QMC) simulations ( Fig. 3 ). As these simulations agree very well with the measurements, they inspire further confidence in the accuracy of the DFT-based values. Table 1 Microscopic model parameters from density functional theory (DFT). 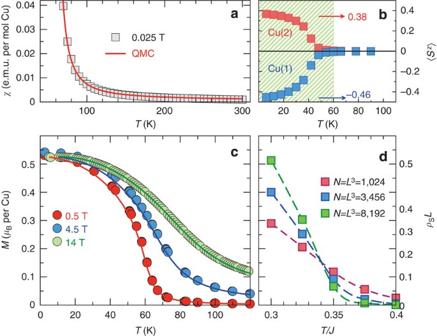Figure 3: Comparison to thermodynamic data. (a) Experimental susceptibilityχ(T) (squares, data evaluted from 1/χdependence in Fig. 4a of ref.20) in comparison with Quantum Monte Carlo (QMC) simulations for the microscopic magnetic model (solid line). (b) QMC simulations for the local spin lengths ‹Sz› of Cu(1) and Cu(2) spins as a function of temperature. The shaded area shows the magnetically ordered region. Arrows indicate the limiting values of the local spin lengths asT→0. (c) Experimental51Tdependence of the magnetization in external magnetic fields of 0.5, 4.5 and 14 Tesla (circles) in comparison with QMC simulations for the microscopic magnetic model (lines). The simulatedχ*(T/J) andM*(T/J) curves are scaled withJ=170 K and the experimentalg=2.11 (ref.21). (d) Finite-size scaling of the spin stiffness for finite lattices up toN=8,192 sites. The crossing pointT/J≃0.34 indicates the ordering temperature. Full size table Figure 3: Comparison to thermodynamic data. ( a ) Experimental susceptibility χ ( T ) (squares, data evaluted from 1/ χ dependence in Fig. 4a of ref. 20 ) in comparison with Quantum Monte Carlo (QMC) simulations for the microscopic magnetic model (solid line). ( b ) QMC simulations for the local spin lengths ‹ S z › of Cu(1) and Cu(2) spins as a function of temperature. The shaded area shows the magnetically ordered region. Arrows indicate the limiting values of the local spin lengths as T →0. ( c ) Experimental [51] T dependence of the magnetization in external magnetic fields of 0.5, 4.5 and 14 Tesla (circles) in comparison with QMC simulations for the microscopic magnetic model (lines). The simulated χ *( T / J ) and M *( T / J ) curves are scaled with J =170 K and the experimental g =2.11 (ref. 21 ). ( d ) Finite-size scaling of the spin stiffness for finite lattices up to N =8,192 sites. The crossing point T / J ≃ 0.34 indicates the ordering temperature. Full size image We emphasize that the calculated J s between Cu(1) and Cu(2) are antiferromagnetic (AFM) and between Cu(2) and Cu(2) ferromagnetic (FM), and so the resulting spin model is not frustrated. The skyrmionic physics stems from the DM interactions, which impair the homogeneity of the FM order parameter and cause a chiral double-twisting of the spins [10] , [11] , [12] . Identification of the basic magnetic building block The exchange integrals ( Table 1 ) reveal a pronounced hierarchy of magnetic energy scales in Cu 2 OSeO 3 . Specifically, there is a striking difference between two groups of exchange couplings, splitting the system into two kinds of Cu 4 tetrahedra: one with strong (| J S |~130–170 K) and the other with weak (| J W |~30–50 K) exchange couplings (see Supplementary Fig. 2 ). Most of the DM terms are much smaller than the isotropic exchange: | D ij | ≪ | J ij |. The four S =1/2 spins of a strong Cu 4 tetrahedron can couple together to form either two total singlets (that is, with total spin S t =0), three triplets ( S t =1) or a quintet state ( S t =2). In a tetrahedron with three AFM and three FM exchange couplings, the ground state (GS) is a total S t =1 triplet, see Fig. 2b,c . The triplet GS is separated from the other spin-multiplets by a large energy gap of ~275 K. An important point is that the Cu 4 tetrahedron triplet wavefunction is not the classical (tensor product) state |↑↑↑ ⇓ › (where the double arrow labels the Cu(1) site in the tetrahedron) but rather a coherent quantum superposition of four classical states with M labelling the three orthogonal triplet states with M =−1, 0, 1 (for brevity, only the M =1 wavefunction is given above). Although these are not the exact tetrahedron basis states due to the presence of a finite triplet-quintet mixing (see methods section), this representation is qualitatively correct. This effective spin wavefunction is consistent with the experimental observation of a locally ferrimagnetic order parameter [20] , [21] . The quantum fluctuations ingrained into these triplet wavefunctions, however, give rise to a substantial reduction of the local moments ( Table 2 ), pinpointing the origin of the small moments observed experimentally [20] . As opposed to transversal spin fluctuations arising from spin waves (which are small [23] , on account of the high dimensionality, the ferrimagnetic nature of the order parameter and the absence of frustration), these local quantum fluctuations are longitudinal in character and hence directly affect the effective magnitude of the spin. This picture is confirmed by a lattice QMC simulation for the full model of Cu S =1/2 spins ( Fig. 3b ). Table 2 Main parameters of the theory. Full size table Not only are the effective triplets responsible for the spin length reduction, they also have a decisive role for several other aspects of direct experimental interest, such as the ordering temperature, the skyrmion diameter and even the sign of the magnetic chirality. The quantum-mechanical nature of the effective triplets is therefore utterly essential, in as much as a simple classical treatment delivers a quantitatively and even qualitatively wrong picture, as becomes clear below. Effective description The above description establishes Cu 4 tetrahedra carrying magnetic triplets as building blocks in Cu 2 OSeO 3 at the next step of the multi-scale approach. Within this abstraction, each of these tetrahedra can be contracted to a single lattice point which, by symmetry, can be chosen to coincide with the position of the corresponding Cu(1) site. The ensuing framework is shaped by corner-shared triangles that together constitute a trillium lattice, which is precisely the same lattice that is formed by the Mn atoms in the B20 structure of MnSi and the Fe atoms in FeGe. This establishes a very close analogy between Mott insulating Cu 2 OSeO 3 and these well-known metallic helimagnets, despite the fundamental differences in electronic structure. However in Cu 2 OSeO 3 , the effective triplet interactions can be derived relying on rigorous microscopic results. At this point both the weaker superexchange couplings J w and the DM interaction D ij become crucial. A straightforward perturbative calculation reveals that their net effect is a weak FM interaction between nearest-neighbour (NN) and next-nearest-neighbour (NNN) tetrahedral entities, with effective exchange couplings ( Table 2 , without spin-mixing) respectively, reflecting the tendency of the system towards FM ordering. This drastic reduction of the energy scale in the effective model is caused by the renormalization of the local spin moments and the sizable quantum fluctuations inside the magnetically strong tetrahedra. Experimentally, the most direct consequence of this energy scale reduction is the value of T C : while a single-site mean-field decoupling in the original spin-1/2 model gives T C =160 K, the corresponding decoupling in the effective spin-1 model gives T C =−4( J 1 + J 2 ) ≃ 65 K, in much better agreement with the experimental value of 60 K (refs 20 , 21 ). Details of these decouplings are provided in Supplementary Methods and Supplementary Fig. 3 . Besides the exchange interactions, also a DM coupling between NN and NNN entities emerges. Crucially, in the GS of a single strong tetrahedron, all diagonal matrix elements of the DM couplings within the tetrahedron vanish by symmetry. The twisting mechanism that causes chiral helimagnetism in Cu 2 OSeO 3 , therefore originates from the effective DM couplings between the strong Cu 4 tetrahedra: these will be the root cause for skyrmions to emerge. Specifically, we find ( Table 2 , wthout spin-mixing), for a representative NN and NNN bond, respectively, while the DM vectors for the remaining bonds follow by symmetry ( Table 3 ). Table 3 Effective couplings for each of the 12 NN and 12 NNN bonds in the effective model. Full size table Description at the mesoscopic level Having established the effective trillium lattice model of Cu 2 OSeO 3 , we now proceed to the long-wavelength magnetic continuum theory that allows us to describe the helimagnetism of Cu 2 OSeO 3 on the mesoscopic scale. To this end, we follow Gnezdilov et al. [24] and rewrite the four tetrahedral entities in each unit cell in terms of four coarse-grained fields, the total spin per site (in the effective model) and three AFM fields , μ =1–3. The energy in the continuum limit then becomes (see Methods section), in units of K: where j ≡8( J 1 + J 2 ), a =8.91113 Å is the lattice constant, and y =0.88557 is a structural parameter. The first term in equation (5) is the exchange energy of the FM ground state. The second line is the standard expression for the elastic and the twisting portion of the energy in cubic crystals. The last two lines are the cross-coupling terms between the FM mode F and the three AFM canting modes L μ . Importantly, this coupling is particularly strong since ξ ∝ J 1,2 . Minimizing equation (5) with respect to L μ gives So the AFM modes follow adiabatically the twisting of the F field, leading to a characteristic AFM indentation of the double-twisted skyrmionic textures ( Fig. 1e,f ). This AFM superstructure will be discussed further below in relation to experiments. Integrating out the AFM canting modes gives the effective energy density for the total magnetization alone: where χ F =3 j +2 κ 2 / j , ′=− ξ 2 /(2 j ), and ′=+ κξ / j . So we find that both and are renormalized by the antiferromagnetic canting. Importantly, ξ 2 / j ∝ J 1,2 , so we expect a large renormalization for the elastic constant . Indeed, we find ( Table 2 , with spin-mixing) ′=−11.19 K, almost two and a half times smaller than =−27.10 K. Intuitively, this reduction can be understood by the AFM nature of the canting modes which disrupts the dominant FM correlations. Turning to the twisting parameter, we find ( Table 2 , with spin-mixing) =1.27 K and ′=−2.46 K. So not only is ′ larger than , but it also has the opposite sign. This means that the canting modes change the magnetic handedness of the system, an important piece of information which can be accessed experimentally (see Discussion). Finally, with the characteristic diameter Λ′ of the double-twisted skyrmion structures being 2 π /| Q ′| (this distance coincides with the helix period in the helical phase [15] ), with wavenumber , the calculated magnetic constants result in a helix period of ( Table 2 , with spin-mixing) Λ′ ≃ 50.89 nm, which is in striking agreement with the experimentally measured [15] value Λ exp ≃ 50 nm. Thus, these numbers give a very satisfactory estimate of the effective chiral DM couplings given that they are describing a weak spin-relativistic exchange effect, which is greatly modified by the complicated internal canting of the spin structure in Cu 2 OSeO 3 . Dzyaloshinskii model To calculate the magnetic phase diagram we need to go one step further and include entropic effects and further anisotropies beyond the DM interactions. In the following, we cast the theory in terms of the total magnetization per volume M ( r )= M sat (0) F , where M sat (0) is the magnetization density in the field-aligned, ferrimagnetic (1/2 plateau) state at T =0. At the atomic level, M sat (0)=4 gμ B / a 3 , where g is the electronic spectroscopic factor of the Cu 2+ ions, while experimentally [16] , the corresponding magnetization is 0.531 μ B per Cu atom, which amounts to M sat (0)=111.348 kA m −1 . The phenomenological free energy density can be decomposed into three contributions, The first contribution f e contains the last two terms of (8) and the Zeeman energy, where H is the internal magnetic field, =− k B ′/ a M sat (0) 2 and = k B exp /( aM sat (0)) 2 , where we readjust the DM parameter so that the experimental helix period Λ exp =4π / is reproduced. The second term of equation (9) holds the anisotropic couplings beyond the DM contributions. For a cubic crystal, the leading terms, describe the exchange anisotropy ′ and the cubic magneto-crystalline anisotropies 1 and 2 . Finally, the third term of equation (9) collects the leading homogeneous free energy terms, which can be written as the usual Landau expansion for the order parameter field M , where is the Curie temperature in the absence of DM couplings or anisotropies. The parameters , α, β, ′, K 1 and 2 can be estimated with a minimum of empirical additional information from experiment in conjunction with QMC data, following the procedure outlined in the Methods section. 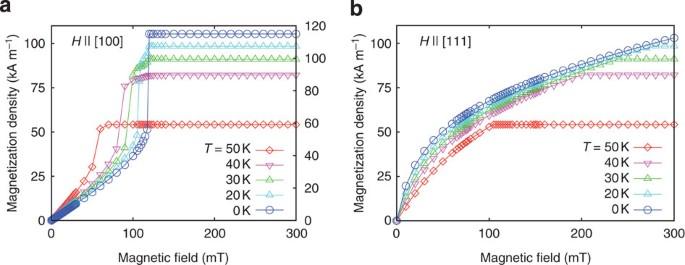Figure 4: Magnetization process of conical helices for the Dzyaloshinskii model. (a) For fields in the easy axis direction [100], the transition to the field-enforced plateau state is discontinuous at a fieldHp(100). (b) For fields in the hard axis direction [111], a continuous transition takes place atHp(111). The resulting estimates are listed in Table 4 . Table 4 Parameters of the Dzyaloshinskii model. Full size table From these parameters we can derive two key quantities of basic experimental interest. The first is the temperature range of the so-called precursor region [12] , [25] , [26] , [27] , where two main effects take place. First, the double-twisted core of skyrmions is energetically favourable and is stabilized at , while the helical ground state sets in only at , and second, the chiral twisting is accompanied by strong longitudinal modulations of the magnetization M . Hence, anomalous skyrmionic spin-textures can be expected within this temperature range. The model parameters yield an estimate Δ T ≃ 1.04 K, in good agreement with the interval of about 2 K in which the so-called ‘A-phases’ appear under magnetic field in Cu 2 OSeO 3 crystals [28] , [29] . Given the crude representation of the thermodynamic potential term in the continuum theory by the Landau expansion, this value gives only the order or magnitude of the expected effects. The second key quantity of interest is the characteristic field strength of the Dzyaloshinskii model, which sets the scale for the unwinding of the chirally twisted helical state into the field-aligned state. With coefficients from Table 4 , a value H D ≃ 0.34 T is found. In turn, this gives the critical field for the closing of the cone state by a continuous spin-flip, H c2 = H D /2 ≃ 0.17 T. Again, these values are in good agreement with experiment (see Methods section). Magnetization process and phase diagram With all this in place, we can fully determine the equilibrium two-dimensional solutions using micromagnetic simulations (see Methods section) [12] , [25] . Figure 4 illustrates the magnetization processes for two different directions of the applied field for constant temperature-depending magnetization . The corresponding characteristic plateau fields H p for the transition between the conical helix and the field-aligned state are shown in Fig. 5a . For fields along [100], the continuous transition from the conical helix state into the field-enforced ferrimagnetic state is found at H c2 ≃ 80 mT at 50 K, in very good agreement with experimental data. Figure 4: Magnetization process of conical helices for the Dzyaloshinskii model. ( a ) For fields in the easy axis direction [100], the transition to the field-enforced plateau state is discontinuous at a field H p (100). ( b ) For fields in the hard axis direction [111], a continuous transition takes place at H p (111). 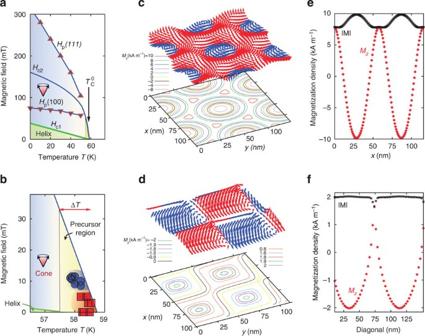Figure 5: Phase diagram from the continuum description of Cu2OSeO3. (a)Hc1denotes the reorientation transition from the helical phase (green region) into the conical state (blue region, indicated by a cone traced by the spins along the propagation direction). Without additional anisotropies, the cone angle closes continuously atHc2and the system reaches the ferrimagnetic plateau phase. A cubic anisotropy makesHc2direction dependent.Hp(111) denotes the continuous transition for fields along [111]. For fields along [100] direction, the conical helix collapses by a first-order process atHp(100). (b) The high-temperature regime of the phase diagram has a narrow precursor region where skyrmionic phases are found numerically for two-dimensional models. Blue circles show the region of stable densely packed ‘’-skyrmion lattices while red squares mark the region of stable ‘’-skyrmion lattices. (c) Magnetization profile of skyrmions. The colouring of the arrows tracks the longitudinal magnetizationMz. The latter is also shown in the projected contour plot with the colouring scheme indicated on the left. (d) Similar tocbut for a half-skyrmion texture. (e) The longitudinal magnetizationMzand the absolute magnetization |M| across two nearest-neighbour (NN) skyrmions ofc. (f) Similar toe, but now we cut across the diagonal of a half-skyrmion texture. Full size image Figure 5: Phase diagram from the continuum description of Cu 2 OSeO 3 . ( a ) H c1 denotes the reorientation transition from the helical phase (green region) into the conical state (blue region, indicated by a cone traced by the spins along the propagation direction). Without additional anisotropies, the cone angle closes continuously at H c2 and the system reaches the ferrimagnetic plateau phase. A cubic anisotropy makes H c2 direction dependent. H p (111) denotes the continuous transition for fields along [111]. For fields along [100] direction, the conical helix collapses by a first-order process at H p (100). ( b ) The high-temperature regime of the phase diagram has a narrow precursor region where skyrmionic phases are found numerically for two-dimensional models. Blue circles show the region of stable densely packed ‘ ’-skyrmion lattices while red squares mark the region of stable ‘ ’-skyrmion lattices. ( c ) Magnetization profile of skyrmions. The colouring of the arrows tracks the longitudinal magnetization M z . The latter is also shown in the projected contour plot with the colouring scheme indicated on the left. ( d ) Similar to c but for a half-skyrmion texture. ( e ) The longitudinal magnetization M z and the absolute magnetization | M | across two nearest-neighbour (NN) skyrmions of c . ( f ) Similar to e , but now we cut across the diagonal of a half-skyrmion texture. Full size image The high-temperature region of the phase diagram is magnified in Fig. 5b to focus on the precursor region close to T C , where skyrmionic cores are energetically more favourable compared with one-dimensional helix solutions [12] , [25] . Here we find two competing skyrmionic phases ( Fig. 5c–f ). The first one ( Fig. 5c,e ) is the standard field-driven ‘− π ’-skyrmion phase of Fig. 1b with the radial skyrmions ordered in a hexagonal lattice [10] , [11] . The second ( Fig. 5d,f ) is the ‘ π /2’-skyrmion state of Fig. 1c , which actually is the stable state at zero and low fields, because the fractionalization of skyrmions into half-skyrmions yields a higher packing density of the energetically advantageous skyrmionic cores. It should be noted that the stability regions of condensed skyrmion phases may be underestimated compared with conical and helicoidal one-dimensional states, as the parallel packing of skyrmionic strings may eventually lower its energy by undergoing a further twisting in the third spatial direction, amounting to a non-trivial conformation of the strings [25] . Furthermore, thermal fluctuations may enhance the stability of skyrmionic phases as they may acquire large configurational entropic contributions compared with the ideal crystalline long-range ordered states, similar to liquids of polymer strings or condensed vortex-matter phases in type-II superconductors. The splitting of defects or of solitonic entities emerges in different research fields [13] , [14] , [30] , [31] , [32] . Yet, for the Dzyaloshinskii models of chiral magnets, a detailed theoretical understanding of the full range of possible textures is still lacking. The main reason is that the splitting of solitons and defect formation relies on a delicate balance between core-energies of solitons and their mutual interactions. In this regard, the emergence of the half-skyrmion phase in the vicinity of the ‘− π ’-skyrmion lattice of Cu 2 OSeO 3 opens a new venue to study the properties of textures with split topological units in experiment. The occurrence of this phase at low fields near the ordering transition should be traceable by thermodynamic measurements revealing further phase transitions in very narrow regions of the precursor range Δ T . Indeed, experimental indications for the presence of more than one mesophase in the precursor region has been reported from macroscopic thermodynamic measurements in the related chiral compounds with B20-structure [26] , [33] , [34] , and in Cu 2 OSeO 3 itself [28] , [35] . Whether one of the phases observed is related to the half-skyrmion phase remains experimentally open, however, and requires further dedicated investigations. To this end, we note that half-skyrmionic phases feature a sizeable longitudinal modulation of the order parameter, and contain defects like hedgehogs or narrow line or wall defects, where the magnetic order parameter M passes through zero. Hence, these textures are expected to display wide distributions of the quasi-static or ordered local magnetic moments, which could be discernible by local probes, such as μ SR and NMR, and used as a signature of the half-skyrmion phase. The defected arrangement of partial skyrmions may also be detected by examining the higher harmonics in the diffraction data. While the finite extension of the radial solitonic cores requires the harmonic contents of a lattice arrangement to display all higher harmonic modes, the dense arrangement of skyrmionic cores and defects in a condensed phase of partial skyrmions will exacerbate these anharmonic effects. Besides the interplay of skyrmion and half-skyrmion phases, the preceding analysis gives several additional important predictions. The first prediction hinges on the observation that the essential magnetic building blocks being weakly coupled, S t =1 tetrahedra has profound ramifications for the magnetic excitation spectrum. It implies that the discrete spin-multiplet excitation spectrum of the four strongly coupled tetrahedron spins (consisting of two total singlets, two triplets and a quintet, see Fig. 2c ) is largely preserved in the translationally invariant system. Therefore, besides the canonical Goldstone mode, a distinct set of weakly dispersive high-energy magnetic excitation modes should appear, where the highest mode goes up to an energy of ~450 K. The detailed form of this structure has been reported by Romhányi et al. [23] , using a fully quantum-mechanical multi-boson expansion. Quite remarkably, this structure was firmly established very recently by Ozerov et al. [36] , using high-field electron spin resonance experiments with a terahertz free electron laser source. The characteristic dispersions associated with the hierarchy of magnetic interactions in Cu 2 OSeO 3 can be further probed by inelastic neutron scattering. The second experimental consequence of the conceptual framework for skyrmion formation in Cu 2 OSeO 3 that we have established here is a canting of the four magnetic sublattices in the trillium lattice. This is similar in spirit to MnSi [37] , but in Cu 2 OSeO 3 the canting must lead to a weakly antiferromagnetic modification of the primary ferrimagnetic order parameter that is related to the long-range ordering of the S t =1 tetrahedron spins. This weak antiferromagnetism in Cu 2 OSeO 3 is the dual counterpart of the weak ferromagnetism that is present in chiral acentric bipartite antiferromagnets [38] . The presence of this antiferromagnetic superstructure implies that in neutron (or resonant x-ray) diffraction experiments there be an additional set of corresponding magnetic Bragg peaks. Establishing their presence experimentally will prove that the skyrmions in Cu 2 OSeO 3 , which have a typical length scale of ~50 nm, carry an extra antiferromagnetic spin-modulation on a length scale more than two orders of magnitude smaller ( Fig. 1e,f ). We have also shown that the canting has a strong influence on the primary order parameter, on account of a sizeable cross-coupling mechanism. Besides the renormalization of the helix period, this coupling actually reverses the magnetic handedness of the system, a key aspect that can be confirmed experimentally with polarized neutrons [39] , [40] , [41] , [42] , [43] , [44] . Indeed, while preparing the final version of our manuscript, we became aware of a new experimental study by Dyadkin et al. [45] , which confirms our theoretical prediction for the sign of the magnetic handedness of Cu 2 OSeO 3 . Choice of enantiomer All our calculations were done for the enantiomer defined by the following crystallographic positions of the Cu sites (in units of the lattice constant a =8.91113 Å): where y =0.88557, a =0.13479, b =0.12096 and c =0.87267. The first four are the Cu(1) sites (Wyckoff positions 4 a ) and the remaining ones are the Cu(2) sites (general 12 b positions). In the convention used in MnSi crystals (with Mn atoms corresponding to Cu(1) atoms in Cu 2 OSeO 3 ), this is the right-handed enantiomer. The positive value of the wavevector Q ′ ( Table 2 ) then means that in Cu 2 OSeO 3 , the magnetic structure displays the same chirality with the crystal structure, in agreement with the new experimental study of Dyadkin et al. [45] Ab initio calculations DFT calculations were performed using fplo version 9.07 (ref. 46 ) based on an extended set of local orbitals and VASP version 5.2 (refs 47 , 48 ) employing the projector-augmented wave method. For DFT calculations, we adopt the experimental structural data from Table 1 of ref. 20 , without performing additional relaxations of unit cell parameters and atomic coordinates. For the exchange and correlation potential, we used the GGA (PBE96) parameterization. The k -meshes were checked for convergence. Relevant couplings ( Supplementary Table 1 ) were evaluated by mapping the GGA band structure ( Supplementary Fig. 4 ) onto the Cu-centered Wannier functions. Isotropic (anisotropic) magnetic exchange couplings were evaluated using scalar-relativistic (full relativistic) spin-polarized DFT+ U total energy calculations, adopting U d =10.5 eV and 9.5 eV for Cu(1) and Cu(2), respectively. Further details on the computational method are provided in Supplementary Methods . QMC simulations QMC simulations of thermodynamical behaviour were done using the code loop from the software package ALPS version 1.3 (ref. 49 ). Simulations were performed on finite lattices of 8,192 spins S =1/2 using periodic boundary conditions, with 40,000 sweeps for thermalization and 400,000 sweeps after thermalization. Triplet-quintet spin-mixing We first summarize the main spectral features of an isolated ‘strong’ tetrahedron. This is described by the spin Hamiltonian (modulo an overall constant), where S 123 is the total spin quantum number of the Cu(2) sites, S 4 is the Cu(1) spin, and S = S 123 + S 4 is the total spin. Thus the spectrum can be labelled by the good quantum numbers | S 12 , S 123 , S , M ›, where M is the total magnetization. The eigenspectrum of 0 ( Fig. 2c ) consists of a ground state triplet |1, 3/2, 1, M ›, two excited singlets |0, 1/2, 0, 0› and |1, 1/2, 0, 0› at energy (measured from from the ground state), a quintet |1, 3/2, 2, M › at and two triplets |0, 1/2, 1, M › and |1, 1/2, 1, M › at . The spin-mixing effect amounts to a finite admixture of the quintet state into the triplet ground state and originates in the weak couplings between the ‘strong’ tetrahedra. To understand this effect, we treat the weak inter-tetrahedral couplings at the mean-field level which, as shown in ref. 23 , is an excellent approximation for the ground state. The resulting ‘tetrahedral mean-field’ (TMF) theory amounts to decoupling the bare S =1/2 model into a sum of independent TMF Hamiltonians with local mean fields acting on the four spins, where ζ and η are self-consistent mean-field parameters, Given that and do not commute with the total spin S , the mean fields admix states with different S . The admixed states must however share the same M and S 123 , which remain good quantum numbers. It follows that the triplet ground state is admixed only with the quintet state. In the M =1 manifold {| φ 1 › ≡ |1, 3/2, 1, 1›,| φ 2 › ≡ |1, 3/2, 2, 1›} we have, apart from an overall constant: Solving self-consistently for the ground state of this matrix leads to the local spin lengths and . Effective model As mentioned above, the effective description of Cu 2 OSeO 3 relies on replacing the magnetically ‘strong’ tetrahedra with effective quantum-mechanical entities, which by symmetry can be placed on the corresponding Cu(1) sites, forming a trillium lattice. For the moment, we disregard the spin-mixing effect, that is, we regard each entity as a faithful spin-1 object (we shall return to this below). The first-order coupling between the effective S t =1 entities can be found using equivalent operators where the spin lengths l 1,2 can be found from (2): l 1 =1/4 and l 2 =5/12. A close inspection of the structure reveals that there are two types of bonds between effective spins and ( Fig. 6 ), one where the tetrahedra t 1 and t 2 are connected via two weak Cu(1)-Cu(2) couplings, and , and another where they are connected via a weak Cu(2)-Cu(2) coupling . 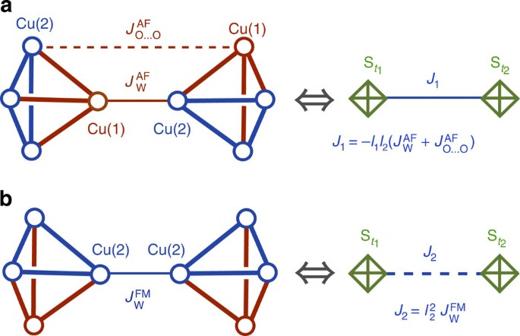Figure 6: Exchange couplings between effective tetrahedral entities. (a) Illustration of how the bare couplingsandof theS=1/2 model give rise to an effective nearest-neighbour (NN) couplingJ1between tetrahedra. The constantsl1andl2are given in the text and depend on whether one includes the spin-mixing effect or not. The spins of the two effective tetrahedra involved in this coupling are denoted byand. In theS=1/2 model, different microscopic couplings are denoted by different line styles, while blue (red) colour generally refers to ferromagnetic (antiferromagnetic) exchange. The couplinginvolves a longer-range O-Se-O super-exchange path along the diagonals of hexagonal loops (here only half of such a loop is visible), which are formed by alternatingbonds (the Se sites reside at the centre of these loops). (b) Similarly for the NNN couplingJ2, where the two tetrahedra are connected via a single bare coupling,. In the trillium lattice, and are, respectively, NN and NNN sites, and the corresponding couplings from first-order perturbation theory are Figure 6: Exchange couplings between effective tetrahedral entities. ( a ) Illustration of how the bare couplings and of the S =1/2 model give rise to an effective nearest-neighbour (NN) coupling J 1 between tetrahedra. The constants l 1 and l 2 are given in the text and depend on whether one includes the spin-mixing effect or not. The spins of the two effective tetrahedra involved in this coupling are denoted by and . In the S =1/2 model, different microscopic couplings are denoted by different line styles, while blue (red) colour generally refers to ferromagnetic (antiferromagnetic) exchange. The coupling involves a longer-range O-Se-O super-exchange path along the diagonals of hexagonal loops (here only half of such a loop is visible), which are formed by alternating bonds (the Se sites reside at the centre of these loops). ( b ) Similarly for the NNN coupling J 2 , where the two tetrahedra are connected via a single bare coupling, . Full size image To check the adequacy of first-order perturbation theory, we have pushed the expansion up to second order. We found that the second-order corrections are , , an order of magnitude weaker than the first-order contributions, and so we can safely disregard them for all practical purposes. For completeness we should also note that in second order there appears an effective bi-quadratic exchange term of the form . The corresponding NN and NNN coefficients are also extremely small ( , ) and can be safely disregarded. Next, we treat the DM couplings, beginning with the ones within the strong tetrahedra, namely and . It turns out that all diagonal matrix elements of these couplings within the ground state triplet manifold vanish by symmetry and so, to lowest order, and do not have any role at all (this remains true with spin-mixing present as well). In other words, the double-twisting mechanism responsible for the appearance of the helical and the skyrmion lattice phase originates in the DM couplings between the strong tetrahedra. The first-order effect of the latter can be treated in exactly the same way as the exchange couplings. Again there are only two independent DM couplings, one for NN and another for NNN bonds of the trillium lattice. By symmetry, we can write all DM couplings in terms of the two vectors of equation (4), see Table 3 . To find the latter, we use Table 3 and proceed as follows. The bond { ρ 1 , ρ 8 } maps to the bond { ρ 1 , ρ 3 +(1,0,0)} in the effective lattice. So, the first-order contribution from to the effective DM vector is . Similarly, the bond { ρ 4 , ρ 12 } maps to { ρ 4 , ρ 2 }, and thus the contribution from to the effective DM vector is . Altogether, Finally, the two Cu(2) sites { ρ 5 , ρ 12 } map to { ρ 1 , ρ 2 +(1,1,0)}, up to a primitive translation. Hence, equals , that is, Let us now incorporate the ground-state spin-mixing effect discussed above. Due to this spin-mixing, the operators S t do not satisfy the commutation relations of spins, but they can still be thought of as vector operators of length one. The first-order perturbation theory in the ground state of equation (19) amounts to simply replacing the local spin lengths and in the above first-order expressions. Table 2 lists the resulting values of various parameters of the model with and without spin-mixing. Continuum limit of the effective model Here we briefly outline the basic steps and assumptions leading to equation (5). Our approach follows the standard route of Taylor expanding the magnetic energy in the long-wavelength limit. Namely, for an effective entity at R + r i , where R labels the Bravais positions in the trillium lattice. In the next step, we express S i ( R ) in terms of F ( R ) and L μ ( R ) (see above), and collect all terms resulting from the 24 exchange and 24 DM anisotropy terms per unit cell, which requires performing a number of lattice summations (see Supplementary Methods , Sec. 4). Next, given that the ferromagnetic mode F is the dominant one, we disregard quadratic terms in L μ , as well as terms of the type a D ij L μ ∂ F or a 2 D ij L μ ∂ 2 F . The latter scale, respectively, as and since , see equation (7). Essentially, this amounts to collecting all energy terms up to . Disregarding unimportant boundary terms then leads to equation (5), which is invariant under the symmetry group P 2 1 3 of the crystal, and in particular under the three-fold rotation around ρ 1 , which takes ( x , y , z ) → ( z , x , y ) in spin space, and ( ρ 2 , ρ 3 , ρ 4 ) → ( ρ 3 , ρ 4 , ρ 2 ) (see coordinates above), or its equivalent form ( F , L 1 , L 2 , L 3 ) → ( F , L 2 , L 3 , L 1 ). The present approach is different from the one followed in ref. 50 for the model on MnSi (which has the same lattice with our effective model). We first remark that in the crystal structure of Cu 2 OSeO 3 , the quantity x ≡1− y =0.11443<1/8, while in MnSi x =0.138>1/8. This means that the second (third) neighbour bonds in Cu 2 OSeO 3 correspond to third (second) neighbour bonds in MnSi (at x =1/8, the two bond types have the same distance). So to apply the results of ref. 50 to our case, we must replace and in the expressions of ref. 50 . With these replacements, the resulting expressions for and are identical with the first two lines of equation (6), but with the important difference that 1− y is replaced by a quantity that depends nonlinearly on the exchange couplings, see ref. 50 for further details. This leads to very different numerical values for and and a helix period Λ ≃ 1514, nm, which is too large compared with the experimental Λ exp =50 nm (ref. 15 ). Parameters of the Dzyaloshinskii model The parameters , α and β ( Table 4 ) were extracted by fitting the mean-field equation of state for the net magnetization M =| M | in the vicinity of the ordering temperature (where the effect of f a can be disregarded, see below), to the QMC data, Fig. 3 , in appropriate ranges 40 K< T <60 K and H <5 T. For the anisotropic parameters of f a , the empirical data from experiment show sizeable and positive 1 , and negligible 2 and ′. This can be seen from the reported [16] anisotropic behaviour of the spin-flip field H c2 , which corresponds to the unwinding of the chirally twisted helical state into the field-aligned state: At temperatures below ~(2/3) , H c2 becomes anisotropic, with the [100]-direction as easy axis and the [111]-direction as hard axis. The splitting between hard and easy axis directions, , reaches ~0.04 T at low temperatures [16] . This behaviour can be qualitatively understood by noting that the effect of 1 sets in when the magnetization tends towards saturation, and if the exchange anisotropy ′ is relatively much smaller (the latter has been checked independently by ab initio calculations at the atomic level). That the value of 1 is sizeable can be also seen by the remarkably high fields H c1 ~0.02–0.035 T (ref. 16 ), corresponding to the helix reorientation transition from the helicoidal states or a multi-domain helix state into the conical helix state, that is, the flopping of the helix in field direction. As the ratio H c2 / H c1 is not small, also the ratio between anisotropy and DM-coupling is expected to be sizeable. One source of 1 comes from the magnetoelectric effect but, as shown in the Supplementary Methods (Sec. 3) based on the experimental magnetoelectric data [16] , this contribution is too small to account for the experimental data. Here, the numerical value of 1 ( Table 4 ) has been adjusted to reproduce the field H c2 in the (100) field direction. The quality of these numbers can be appreciated by a comparison with experiment. Magnetization data on single crystals show that H c2 does not depend significantly on the applied field direction for T >35 K (refs 16 , 29 , 35 ). In this range, we can also use the isotropically averaged magnetization data on polycrystalline samples [20] , which give H c2 ≃ 73 mT at T =50 K. At the same temperature, single crystal magnetization data give estimates H c2 ≃ 68 and 70 mT for fields in [100] and [−554] direction, respectively, after the demagnetization corrections [16] , while magnetization data on another single crystal gives H c2 ≃ 60, 58 and 56 mT for field directions [100], [110] and [111], respectively [35] . Other data by Adams et al. [29] report higher values (ref. 29 ), while Seki et al. [15] report . Some of the deviations may be traced back to demagnetization corrections, but the model is seen to be in reasonable agreement with the experimental facts. Micromagnetic calculations The determination of equilibrium states for the completed Dzyaloshinskii continuum model requires energy minimization of the free energy density functional of equation (9). The calculation of modulated states including the cubic anisotropy with coefficient K 1 as given in Table 4 has been performed by numerical micromagnetic calculations using finite difference discretization with adjustable grid spacings and periodic boundary conditions. Energy minimization used simulated annealing for the search of initial solutions and a relaxation and grid refinement. In this way, two-dimensional equilibrium solutions have been calculated (In Fig. 5 , the ‘− π ’-Skyrmion lattice is the solution for H =7 mT and T =58.1 K, while the ‘ π /2’-lattice is the solution for H =4 mT and T =58.7 K.) These solutions are constrained approximations to three-dimensional textures composed of skyrmionic strings, as they represent states with homogeneous spin structure in the third spatial direction. How to cite this article : Janson, O. et al. The quantum nature of skyrmions and half-skyrmions in Cu 2 OSeO 3 . Nat. Commun. 5:5376 doi: 10.1038/ncomms6376 (2014).